COG complexes form spatial landmarks for distinct SNARE complexes Vesicular tethers and SNAREs (soluble N-ethylmalemide-sensitive fusion attachment protein receptors) are two key protein components of the intracellular membrane-trafficking machinery. The conserved oligomeric Golgi (COG) complex has been implicated in the tethering of retrograde intra-Golgi vesicles. Here, using yeast two-hybrid and co-immunoprecipitation approaches, we show that three COG subunits, namely COG4, 6 and 8, are capable of interacting with defined Golgi SNAREs, namely STX5, STX6, STX16, GS27 and SNAP29. Comparative analysis of COG8-STX16 and COG4-STX5 interactions by a COG-based mitochondrial relocalization assay reveals that the COG8 and COG4 proteins initiate the formation of two different tethering platforms that can facilitate the redirection of two populations of Golgi transport intermediates to the mitochondrial vicinity. Our results uncover a role for COG sub-complexes in defining the specificity of vesicular sorting within the Golgi. The transport of vesicular carriers in the secretory pathway is a multistep process that includes vesicle budding, tethering, docking and fusion [1] . Vesicle tethering, the initial contact between an intracellular trafficking vesicle and its membrane target, requires the participation of both long coiled-coil tethers and multi-subunit hetero-oligomeric tethering complexes (MTCs) [2] . Tethering complexes, in concert with small Rab GTPases, Sec1/Munc18(SM) proteins and SNAREs (soluble N-ethylmalemide-sensitive fusion attachment protein receptors), regulate the docking of a vesicle to its acceptor compartment, and thereby determine the targeting specificity of vesicles. Such targeting is a critical determinant of protein sorting, and thus maintaining the compartmental identity within the secretory pathway. MTCs form a group of large evolutionary conserved peripheral protein complexes that function throughout the secretory pathway. Included within this superfamily of proteins is a family termed CATCHR (complexes associated with tethering containing helical rods) that consist of the conserved oligomeric Golgi (COG) complex, the Golgi-associated retrograde protein complex (GARP), the Exocyst complex and the Dsl1 complex [3] . Multiple modes of interaction between MTCs and other components of the vesicle docking/fusion machinery have recently been suggested [4] , [5] , [6] , [7] . The COG complex consists of eight subunits named COG1–8 ( [8] , [9] ), grouped into two sub-complexes: COG1–4 (Lobe A) and COG [5] , [6] , [7] , [8] (Lobe B) [10] , [11] . The COG complex functions in the tethering of vesicles recycling resident Golgi proteins (such as glycosylation enzymes) [12] . Consequently, defects in COG complex subunits result in congenital disorders of glycosylation type II [13] . We have shown previously that the yeast and mammalian COG complex interacts with the Sed5/STX5-containing SNARE complex [14] , [15] through a direct interaction between COG4 and Sed5/STX5. Interference with this interaction results in a decreased steady-state level of intra-Golgi SNARE complexes. In this study, we have extended our initial investigation of COG–SNARE interactions to include 14 known Golgi-localized SNARE proteins and all COG subunits. Our results demonstrate specific interactions of COG4, 6 and 8 with the five Golgi SNAREs STX5, STX6, STX16, GS27 and SNAP29 by yeast two-hybrid and native co-immunoprecipitation (co-IP) approaches. A mitochondrial COG relocalization assay revealed a unique feature of COG–SNARE interactions, with COG4 mislocalization redirecting STX5-containing vesicles, and COG8 mislocalization redirecting STX16-containing membranes to COG-occupied mitochondria. Our results indicate that one of the major functions of COG sub-complexes is to serve as landmarks for the initiation of tethering platforms for at least two different types of intra-Golgi vesicles. COG complex interacts with multiple Golgi SNAREs To uncover the complete set of COG–SNARE interactions, we performed a directed yeast two-hybrid screen of all eight COG subunits with 14 Golgi-localized SNARE proteins. 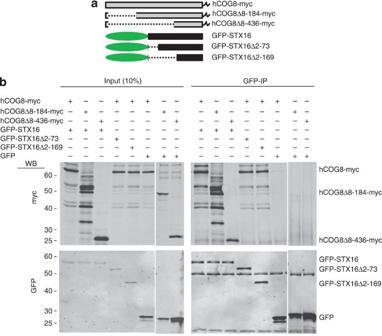Figure 1: COG8 C terminus interacts with SNARE domain of STX16. HeLa cells transiently co-transfected with plasmids encoding fluorescent-tagged SNAREs and COG-myc constructs as indicated (a). 24 h post transfection, cells were collected and lysed, and GFP–SNARE-interacting proteins were precipitated with anti-GFP antibodies. Immuno-precipitates, along with 10% of total input, were separated on a 12% SDS–PAGE gel, transferred to nitrocellulose membrane and probed with antibodies against myc (b, upper panel) and GFP (b, lower panel). COG8Δ8-184-myc and COG8Δ8-436-myc are still capable of interaction with full-length GFP-STX16. GFP-STX16-truncated mutants missing either the N terminus (GFP-STX16 Δ2-73) or N terminus and Habc domain (GFP-STX16 Δ2-169) are both still capable of interaction with full-length COG8-myc. Of these, only the Qa SNAREs STX5 and STX16, the Qb SNARE GS27, the Qc SNARE STX6 and the Qab SNARE SNAP29 displayed positive interactions with subunits of the COG complex ( Table 1 and Supplementary Fig. S1 ). Similarly, only a subset of the COG subunits, namely COG4, 6 and 8, displayed an interaction with SNAREs. As previously reported [15] , COG4 demonstrated a unique interaction with STX5 under strong selection (-Ade). COG6, in addition to previously reported interactions with STX5 (ref. 15 ) and STX6 (ref. 16 ), also specifically interacted with GS27 and SNAP29. Finally, COG8 displayed a novel set of interactions with the SNAREs STX5, STX6, STX16 and GS27; of these, STX5, STX16 and GS27 were observed under stringent selection conditions ( Table 1 and Supplementary Fig. S1 ). The observed yeast two-hybrid interactions were validated in co-IP experiments ( Supplementary Fig. S2 ). Table 1 SNAREs interact with COG4, COG6 and COG8 subunits. Full size table To further characterize the novel interaction between COG8 and STX16, we constructed truncated mutants of both COG8-myc (based on predicted breaks in the alpha-helical domains) and green fluorescent protein (GFP)-STX16 (at known domain boundaries) ( Fig. 1a ), and tested them for interaction by co-IP. COG8-mycΔ8-184 was immunoprecipitated as efficiently by GFP-STX16 as full-length COG8-myc, indicating that the COG8 N-terminal domain is dispensable for the COG8-STX16 interaction. Significant co-IP (4%) was also observed for the STX16-COG8-mycΔ8-436 pair, indicating that the C-terminal domain of COG8 is partially sufficient for the interaction with STX16 ( Fig. 1b , lanes 1–3). Furthermore, truncated mutants of GFP-STX16 reveal that both the N-terminal (amino acid (aa) 2–73) and the Habc (aa 73–169) domains of STX16 are dispensable for the COG8-STX16 interaction, indicating that the C-terminal SNARE domain-containing region of STX16 is the major binding partner of COG8 ( Fig. 1b , lanes 4–6). Figure 1: COG8 C terminus interacts with SNARE domain of STX16. HeLa cells transiently co-transfected with plasmids encoding fluorescent-tagged SNAREs and COG-myc constructs as indicated ( a ). 24 h post transfection, cells were collected and lysed, and GFP–SNARE-interacting proteins were precipitated with anti-GFP antibodies. Immuno-precipitates, along with 10% of total input, were separated on a 12% SDS–PAGE gel, transferred to nitrocellulose membrane and probed with antibodies against myc ( b , upper panel) and GFP ( b , lower panel). COG8Δ8-184-myc and COG8Δ8-436-myc are still capable of interaction with full-length GFP-STX16. GFP-STX16-truncated mutants missing either the N terminus (GFP-STX16 Δ2-73) or N terminus and Habc domain (GFP-STX16 Δ2-169) are both still capable of interaction with full-length COG8-myc. Full size image COG targeting to mitochondria causes relocalization of Golgi markers To gain a better understanding of the nature and hierarchy of COG–SNARE interactions, a mitochondrial mislocalization strategy [17] was employed. Small interfering RNA (siRNA)-resistant COG complex subunits were fused to mCherry fluorescent protein and the mitochondrial-targeting ActA sequence from Listeria ( Fig. 2a ). Transient expression of mCherry-ActA (mChActA) demonstrated intense labelling of the mitochondrial network without any visible effect on Golgi or mitochondrial structure ( Fig. 2b ). Surprisingly, expression of either COG8-mChActa ( Fig. 2c ) or COG4-mChActA ( Fig. 2e ) caused dramatic changes to both Golgi and mitochondrial morphology. Both immunofluorescence (IF) ( Fig. 2b–e ) and electron microscopy (EM) ( Fig. 2f ) approaches revealed that in cells expressing either COG8-mChActa or COG4-mChActA, the majority of the mitochondria were aggregated, whereas Golgi membranes were severely fragmented ( Fig. 2l ). Importantly, aggregation of the mitochondria was not the result of possible cross-linking via COG8 or COG4 self-dimerization, because these subunits did not show any potency for self-dimerization in either yeast two-hybrid or mammalian-expression assays [11] . Overexpression of COG4-myc partially alleviated the COG4-mChActA-induced mitochondrial aggregation ( Supplementary Fig. S3 ), possibly by competing for the additional proteins and/or membranes responsible for this aggregation. 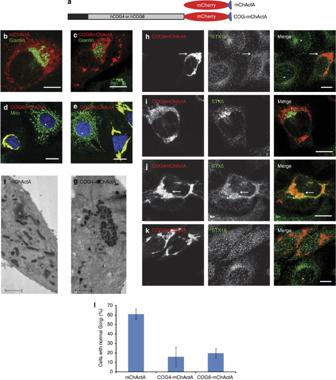Figure 2: Mitochondrial clustering and Golgi fragmentation in cells expressing COG subunits on mitochondria. A schematic diagram of the mitochondrial-targeting protein constructs (a). HeLa cells expressing mChActA (b,f), COG8-mChActA (c,d) or COG4-mChActA (e,g) were analysed 24 h after transfection using confocal or TEM microscopy. Cells were stained with antibodies to Giantin (b,c) to identify Golgi, or mitochondria-resident protein Ox Phos ComplexV (d,e) to image mitochondria. Mitochondria are not clustered in untransfected cells (d,e, asterisk), or in cells expressing mChActA (b,f), and clustered in cells expressing COG8-mChActA (c,d) or COG4-mChActA (e,g). Using a gene-replacement strategy, cells were depleted of COG8 (h,i) or COG4 (j,k) using siRNA transfection. Seventy-two hours after knockdown, cells were transfected with siRNA-resistant COG8-mChActA (h,i) or COG4-mChActA (j,k), and 24 h later, cells were stained with antibodies to STX16 (h,k) or STX5 (i,j) (asterisk denotes non-transfected cell). Endogenous STX16 is partially mislocalized to COG8-labelled mitochondria (h), whereas endogenous STX5 shows co-localization with COG4-clustered mitochondria (j). Quantification of the Golgi disruption phenotype in cells expressing mitochondria-targeted COG subunits (l). HeLa cells plated on coverslips were transfected with plasmids encoding either mChActA, COG4-mChActA or COG8-mChActA. Twenty-four hours after transfection, cells were fixed and stained with antibodies against GM130 and analysed using confocal microscopy. Scale bars, IF 10 μm, TEM 2 μm. Golgi fragmentation was scored by evaluation of Golgi morphology based on GM130 signal in transfected cells. Averages of three independent measurements, mChActAn=66, COG4-mChActAn=44, COG8-mChActAn=38. Error bars denote s.d. from average. Figure 2: Mitochondrial clustering and Golgi fragmentation in cells expressing COG subunits on mitochondria. A schematic diagram of the mitochondrial-targeting protein constructs ( a ). HeLa cells expressing mChActA ( b , f ), COG8-mChActA ( c , d ) or COG4-mChActA ( e , g ) were analysed 24 h after transfection using confocal or TEM microscopy. Cells were stained with antibodies to Giantin ( b , c ) to identify Golgi, or mitochondria-resident protein Ox Phos ComplexV ( d , e ) to image mitochondria. Mitochondria are not clustered in untransfected cells ( d , e , asterisk), or in cells expressing mChActA ( b , f ), and clustered in cells expressing COG8-mChActA ( c , d ) or COG4-mChActA ( e , g ). Using a gene-replacement strategy, cells were depleted of COG8 ( h , i ) or COG4 ( j , k ) using siRNA transfection. Seventy-two hours after knockdown, cells were transfected with siRNA-resistant COG8-mChActA ( h , i ) or COG4-mChActA ( j , k ), and 24 h later, cells were stained with antibodies to STX16 ( h , k ) or STX5 ( i , j ) (asterisk denotes non-transfected cell). Endogenous STX16 is partially mislocalized to COG8-labelled mitochondria ( h ), whereas endogenous STX5 shows co-localization with COG4-clustered mitochondria ( j ). Quantification of the Golgi disruption phenotype in cells expressing mitochondria-targeted COG subunits ( l ). HeLa cells plated on coverslips were transfected with plasmids encoding either mChActA, COG4-mChActA or COG8-mChActA. Twenty-four hours after transfection, cells were fixed and stained with antibodies against GM130 and analysed using confocal microscopy. Scale bars, IF 10 μm, TEM 2 μm. Golgi fragmentation was scored by evaluation of Golgi morphology based on GM130 signal in transfected cells. Averages of three independent measurements, mChActA n =66, COG4-mChActA n =44, COG8-mChActA n =38. Error bars denote s.d. from average. Full size image Next, we used a gene-replacement strategy to test the localization of Golgi Qa SNAREs in cells that carry only the mitochondria-localized COG subunits. STX16 demonstrated a punctate localization in COG8-deficient cells, and these STX16-positive vesicles were concentrated in the vicinity of COG8-mChActA-aggregated mitochondria ( Fig. 2h , arrow). This pattern was specific for STX16 (and distinct from its WT localization ( Supplementary Fig. S4a )) because endogenous STX5 was mostly excluded from the area occupied by COG8-mChActA-positive mitochondria ( Fig. 2i ). In dramatic contrast, STX5 showed significant co-localization with the COG4-mChActA signal ( Fig. 2j , arrow), whereas STX16 was mostly excluded from the vicinity of COG4-mChActA-aggregated mitochondria ( Fig. 2k ). Because both STX5 and STX16 are transmembrane proteins, their co-localization with COG-decorated mitochondria indicates the relocalization of SNARE-containing vesicles to the mitochondria vicinity. In summary, gene-replacement/relocalization experiments revealed that localization of the endogenous STX16-containing membranes is sensitive to the location of COG8, whereas STX5 ones are sensitive to the intracellular location of COG4. Expression of COG6-mChActA resulted in some mitochondrial aggregation but did not affect either Golgi morphology or localization of Golgi SNARE proteins, and therefore COG6-mChActA was investigated separately [18] . To accurately quantify the COG4-mChActA-induced relocalization of STX5-containing vesicles to mitochondria, we transiently expressed fluorescently tagged STX5 in HeLa cells. Line plot analysis and Pearson’s correlation coefficient demonstrated extensive co-localization of GFP-STX5-containing vesicles with COG4-labelled mitochondria ( Fig. 3b ), validating our results seen with the endogenous protein. In contrast, GFP-STX16 membranes did not move towards COG4-mChActA-populated mitochondria ( Fig. 3d ), indicating that the relocalization of GFP-STX5 vesicles was specific for COG4. Some relocalization to the mitochondria was observed for the STX5 intra-Golgi partner SNARE proteins GS28 and GS27 ( Fig. 3g and Supplementary Fig. S5a,b ), whereas the endoplasmic reticulum (ER)–Golgi SNAREs Bet1 and Sec22 were negative for co-localization to COG4-labelled mitochondria ( Fig. 3g and Supplementary Fig. S5c,d ). Similarly, COG4-dependent relocalization of STX5 vesicles to mitochondria was observed in cells that stably express GFP-STX5 on the Golgi ( Supplementary Fig. S6 ) and in cell fusion experiments ( Supplementary Figs S7 and S8 ), indicating that de novo synthesis of Golgi SNARE molecules is dispensable for their relocalization and that STX5-containing vesicles are re-routed to the mitochondria vicinity directly from the Golgi region. 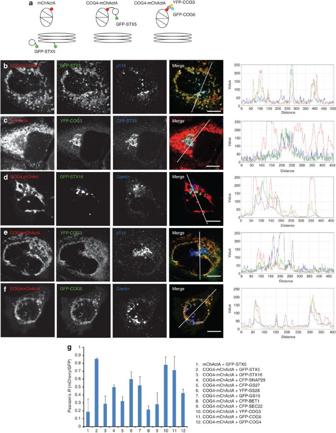Figure 3: Mitochondria-targeted COG4 relocates STX5 membranes and attracts Lobe A and B COG subunits. A schematic diagram of the mitochondrial-targeting protein constructs (a). HeLa cells transiently expressing GFP-STX5 (b), CFP-STX5 (c) and GFP-STX16 (d), or stably expressing YFP-COG3 (c,e) or GFP-COG6 (f), were transfected with a plasmid encoding either mChActA (c) or COG4-mChActa (b,d–f). Twenty-four hours after transfection, cells were fixed, and then stained with antibodies to Giantin or p115 as indicated, and analysed by confocal microscopy. Line plots for overlap between red, green and blue channels are shown measuring the relative value of signal intensity (y-axis) over the distance measured in pixels (x-axis). Scale bar, 10 μm. Plot for the average Pearson’s coefficient for co-localization between mCherry/red and GFP/green signal for indicated constructs and proteins (g). Error bars represent s.d.,n≥3. Figure 3: Mitochondria-targeted COG4 relocates STX5 membranes and attracts Lobe A and B COG subunits. A schematic diagram of the mitochondrial-targeting protein constructs ( a ). HeLa cells transiently expressing GFP-STX5 ( b ), CFP-STX5 ( c ) and GFP-STX16 ( d ), or stably expressing YFP-COG3 ( c , e ) or GFP-COG6 ( f ), were transfected with a plasmid encoding either mChActA ( c ) or COG4-mChActa ( b , d – f ). Twenty-four hours after transfection, cells were fixed, and then stained with antibodies to Giantin or p115 as indicated, and analysed by confocal microscopy. Line plots for overlap between red, green and blue channels are shown measuring the relative value of signal intensity (y-axis) over the distance measured in pixels (x-axis). Scale bar, 10 μm. Plot for the average Pearson’s coefficient for co-localization between mCherry/red and GFP/green signal for indicated constructs and proteins ( g ). Error bars represent s.d., n ≥3. Full size image COG4 interacts physically not only with STX5, but also with its partner protein Sly1 [19] . Interestingly, the COG4(E53A, E71A)- mChActA double mutant, which does not interact with Sly1p, was not capable of attracting GFP-STX5 vesicles ( Supplementary Fig. S9 ), indicating that the functional STX5–Sly1 complex is essential for the movement and/or tethering of STX5 vesicles to COG4-mitochondria. To test if displacement of COG4 to the mitochondria would influence the localization of other COG subunits, we transfected COG4-mChActA into cell lines stably expressing yellow fluorescent protein (YFP)-COG3 ( Fig. 3e ) or GFP-COG6 ( Fig. 3f ). Both YFP-COG3 and GFP-COG6 became significantly co-localized with COG4-mChActA-labelled mitochondria. Similar results were obtained with both myc-COG2 and COG8-GFP ( Supplementary Fig. S10 ), indicating that the entire COG complex relocalized to the COG4-decorated mitochondria. Native IP experiments confirmed that a significant fraction of both myc-COG2 (Lobe A subunit) and COG6-myc (Lobe B subunit) was specifically recovered in COG4-mChActA IP ( Supplementary Fig. S11 ), indicating that the entire COG complex is assembled on the mitochondrial membrane. This relocalization was specific for COG subunits because the cis -Golgi-resident proteins p115 ( Fig. 3b ) and Giantin ( Fig. 3d ) remained associated with fragmented Golgi membranes. Disrupting the interaction of lobes A and B, either by overexpressing a C-terminal fragment of COG1 or by knocking down the COG1 subunit ( Supplementary Fig. S12 ), significantly diminished the relocalization of GFP-STX5 to the COG4-populated mitochondrial membranes, suggesting that the assembly of the functional COG complex on mitochondria is essential for relocalization of STX5-bearing vesicles. Our protein–protein interaction data ( Table 1 and Supplementary Fig. S1 ) indicated that STX5 can bind the COG8 protein to the same or even greater extent as COG4; therefore, we expected that GFP-STX5-bearing vesicles would be relocalized to COG8-decorated mitochondria. To our surprise, in cells that express COG8-mChActA, GFP-STX5 mostly localized to perinuclear fragmented Golgi membranes ( Fig. 4b ), indicating that COG8 alone is not sufficient to attract STX5-containing trafficking intermediates. In contrast, the GFP-STX16 signal was significantly co-localized with COG8-mChActA-decorated mitochondria ( Fig. 4c ), indicating that the STX16-bearing trafficking intermediates become re-routed from the Golgi to another cellular location (presumably to the organelle possessing the highest concentration of COG8 protein). Rapid relocalization of STX16 vesicles to mitochondria was observed in cell fusion experiments ( Supplementary Fig. S13 ), indicating that de novo synthesis of this Golgi SNARE molecule is dispensable for its relocalization and that STX16-containing vesicles were re-routed to mitochondria directly from the trans -Golgi (TGN) region and/or endosomal compartment. 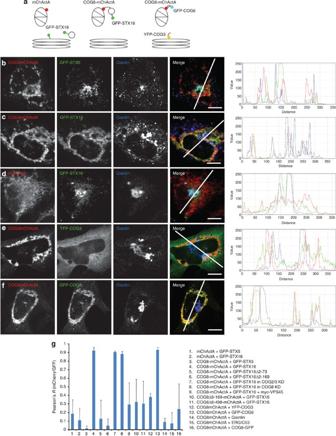Figure 4: Mitochondria-targeted COG8 relocates STX16 vesicles and attracts Lobe B COG subunits. A schematic diagram of the mitochondrial-targeting protein constructs (a). HeLa cells transiently expressing GFP-STX5 (b) and GFP-STX16 (c,d), or stably expressing YFP-COG3 (e) or GFP-COG6 (f), were transfected with a plasmid encoding either mChActA (d) or COG8-mChActa (b,c,e,f). Twenty-four hours after transfection, cells were fixed, stained with antibodies to Giantin and analysed by confocal microscopy. Line plots for overlap between red, green and blue channels are shown measuring the relative value of signal intensity (y-axis) over the distance measured in pixels (x-axis). Scale bar, 10 μm. Plot for the average Pearson’s coefficient for co-localization between mCherry/red and GFP/green signal for the indicated constructs and proteins (g). Error bars represent s.d.,n≥3. Figure 4: Mitochondria-targeted COG8 relocates STX16 vesicles and attracts Lobe B COG subunits. A schematic diagram of the mitochondrial-targeting protein constructs ( a ). HeLa cells transiently expressing GFP-STX5 ( b ) and GFP-STX16 ( c , d ), or stably expressing YFP-COG3 ( e ) or GFP-COG6 ( f ), were transfected with a plasmid encoding either mChActA ( d ) or COG8-mChActa ( b , c , e , f ). Twenty-four hours after transfection, cells were fixed, stained with antibodies to Giantin and analysed by confocal microscopy. Line plots for overlap between red, green and blue channels are shown measuring the relative value of signal intensity (y-axis) over the distance measured in pixels (x-axis). Scale bar, 10 μm. Plot for the average Pearson’s coefficient for co-localization between mCherry/red and GFP/green signal for the indicated constructs and proteins ( g ). Error bars represent s.d., n ≥3. Full size image Co-expression of COG8-mChActA and YFP-COG3 ( Fig. 4e ) revealed that YFP-COG3 did not relocalize to mitochondria, indicating that the Lobe A subunits of COG did not follow COG8. In contrast, GFP-COG6 ( Fig. 4f ) was faithfully recruited to COG8-occupied mitochondria. Because COG6 interacts with COG8 only in the presence of other Lobe B subunits [11] , our results suggest that Lobe B, in its entirety, assembles onto outer mitochondrial membranes decorated with COG8-mChActA. In agreement with this, native IP experiments confirmed that COG6-myc was specifically recovered in a COG8-mChActA IP, whereas myc-COG2 recovery was at background level ( Supplementary Fig. S11 ), indicating that Lobe A subunits are excluded from COG8-decorated mitochondrial membranes. This result is in a good agreement with both previously published, and our recent unpublished data, indicating that approximately 10% of cytoplasmic [9] and 40% of membrane-bound Lobe B exists as the Lobe A-independent sub-complex (Willett, Lupashin; in preparation). As demonstrated above, STX16 is a major SNARE partner of COG8; therefore, we reasoned that direct protein–protein interactions could be the major driving force behind the GFP-STX16 relocalization to mitochondria. To examine this possibility, two truncated mutants of COG8 were tested for their ability to redirect trafficking of GFP-STX16-containing vesicles to mitochondria. Both truncated mutants were capable of binding STX16, as demonstrated by native co-IP ( Fig. 1b ), but failed to redirect STX16 transport intermediates to mitochondria ( Fig. 4g ), suggesting that the direct COG8-STX16 protein–protein interaction is not sufficient to attract STX16-containing vesicles to a new cellular location. Similarly, two truncated mutants of STX16 were not diverted to the COG8-populated mitochondria ( Fig. 4g ), suggesting that only vesicles bearing functional (full-length) STX16 are capable of following fully active COG8 to mitochondrial membranes. The STX16 relocalization appeared to be independent from Lobe A of the COG complex; interaction of STX16 membranes with COG8-mitochondria was not disturbed in cells depleted of COG2 and COG3 proteins ( Fig. 4g ). Endogenous COG8 was also dispensable for the relocalization of STX16 vesicles to COG8-mChActA-populated mitochondria ( Fig. 4g ). Finally, we found that redirection of STX16 vesicles to mitochondria was severely disturbed in cells that overexpress the STX16 partner protein Vps45 ( Fig. 4g ). This suggests that movement of STX16 vesicles to mitochondria recapitulates a bona fide membrane transport step, with COG8 serving as a specific spatial landmark for these STX16-trafficking intermediates. To further investigate the nature of the interaction between COG8-populated mitochondria and STX16-trafficking intermediates, we performed a fluorescence recovery after photobleaching assay with cells that co-express COG8-mChActA and GFP-STX16 ( Fig. 5 ). We found that recovery of GFP-STX16 signal in a bleached area was relatively fast in comparison with the recovery of the mCherry signal, showing that STX16 vesicles are rapidly exchanging on COG8-mitochondria. This indicates that the Lobe B tethering machinery alone is not sufficient for the tight docking of STX16 transport carriers. Furthermore, these results may also indicate that tethering interactions are transient, and that there is a built-in timer that aborts tethering if fusion does not follow. 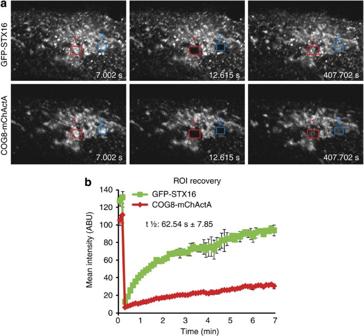Figure 5: GFP-STX16-containing membranes cycle rapidly on/off COG8-mChActA-labeled mitochondria. HeLa cells transiently expressing COG8-mChActA and GFP-STX16 were incubated at 37 °C and visualized with a LSM 710 laser confocal microscope. Both COG8-mChActA and GFP-STX16 were bleached and their fluorescence recovery after photobleaching (FRAP) was measured over a course of 7 min. Representative frames for pre-bleached and post-bleached time points are shown (a). FRAP of COG8-mChActA was slower compared with GFP-STX16, which had at1/2of 62.54 s (b), average from two experiments. ROI, regions of interest. Figure 5: GFP-STX16-containing membranes cycle rapidly on/off COG8-mChActA-labeled mitochondria. HeLa cells transiently expressing COG8-mChActA and GFP-STX16 were incubated at 37 °C and visualized with a LSM 710 laser confocal microscope. Both COG8-mChActA and GFP-STX16 were bleached and their fluorescence recovery after photobleaching (FRAP) was measured over a course of 7 min. Representative frames for pre-bleached and post-bleached time points are shown ( a ). FRAP of COG8-mChActA was slower compared with GFP-STX16, which had a t 1/2 of 62.54 s ( b ), average from two experiments. ROI, regions of interest. Full size image Transmission EM (TEM) was employed for a detailed analysis of STX5- and STX16-containing trafficking intermediates that move to mitochondrial membranes in response to relocalization of COG subunits. Low resolution TEM images ( Fig. 2f ) confirmed that in cells expressing high levels of COG4-mChActA, the mitochondria were mostly found in aggregates. At higher magnification, both membrane tubules and multiple vesicle profiles (arrows) were observed in close proximity to COG4-mChActA- ( Fig. 6a ) and COG8-mChActA- ( Fig. 6b ) populated mitochondria. Vesicles adjacent to mitochondria were uniform in size (60–80 nm), and often connected to the outer mitochondrial membranes by string-like structures ( Supplementary Fig. S14 ) that likely represent protein tethers, such as the COG complex and/or COG-associated proteins. Similar fibrous elements that link vesicle profiles to larger membranes were described previously for vesicles tethered to Golgi cisternae [20] . Immuno-EM with anti-GFP antibodies confirmed that vesicles located in close proximity to (and often in-between) mitochondria were carrying GFP-STX5 ( Fig. 6c ) and GFP-STX16 ( Fig. 6d ). In contrast, in cells that expressed mChActA and GFP-tagged SNAREs, the GFP signal was mostly localized to the Golgi ( Fig. 6e ). 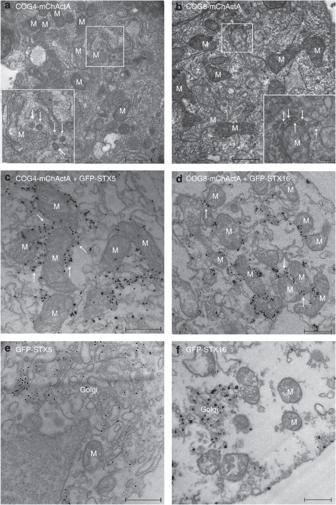Figure 6: Vesicles associate with mitochondria in cells expressing COG8 or COG4 targeted to mitochondria. Electron micrograph of HeLa (a,b) and Vero (c–f) cells transiently transfected with COG4-mChActa (a), COG8-mChActA (b), COG4-mChActA+GFP-STX5 (c), COG8-mChActA+GFP-STX16 (d), mChActA+GFP-STX5 (e) and mChActA+GFP-STX16 (f). Twenty-four hours after transfection, cells were fixed and processed for TEM (a,b) or immuno-EM (c–f). The inset shows a high magnification view of vesicular profiles. Mitochondria (M) and mitochondria-associated vesicles (see arrows) are indicated. Scale bar, 500 nm (inset 100 nm). Figure 6: Vesicles associate with mitochondria in cells expressing COG8 or COG4 targeted to mitochondria. Electron micrograph of HeLa ( a , b ) and Vero ( c – f ) cells transiently transfected with COG4-mChActa ( a ), COG8-mChActA ( b ), COG4-mChActA+GFP-STX5 ( c ), COG8-mChActA+GFP-STX16 ( d ), mChActA+GFP-STX5 ( e ) and mChActA+GFP-STX16 ( f ). Twenty-four hours after transfection, cells were fixed and processed for TEM ( a , b ) or immuno-EM ( c – f ). The inset shows a high magnification view of vesicular profiles. Mitochondria (M) and mitochondria-associated vesicles (see arrows) are indicated. Scale bar, 500 nm (inset 100 nm). Full size image COG8-mChActA misdirects Shiga toxin transporting vesicles to mitochondria We, and others, demonstrated previously that both the COG complex [16] , [21] and STX16 (ref. 22 ) are essential for the intracellular delivery of Shiga toxin from the endosomal compartment to the Golgi. To test if redirection of STX16 vesicles to the COG8-populated mitochondria affects the delivery of Shiga toxin, cells co-expressing COG8-mChActA and GFP-STX16 were pulsed with fluorescent Shiga toxin B subunit (STB-647), and then chased for 2 h in fresh media. In COG8-mChActA-expressing cells, the majority of GFP-STX16 and STB-647 were accumulated in close proximity to mitochondria, suggesting that endosome-to-Golgi-trafficking intermediates that carry STB-647 and GFP-STX16 are redirected to the COG8-mChActA-populated mitochondrial membranes ( Fig. 7a ). In control cells co-expressing mChActA and GFP-STX16, the majority of STB-647 was found in the perinuclear area ( Fig. 7b ), confirming the role of COG8 in determining the fate of STB-647-containing TGN vesicles. Accordingly, trafficking of another COG-dependent toxin, SubAB [23] , was also found to be sensitive to the localization of COG8; a significant fraction of SubAB-647-containing vesicles was redirected to mitochondria in cells that co-express COG8-mChActA and GFP-STX16 ( Supplementary Fig. S15 ). 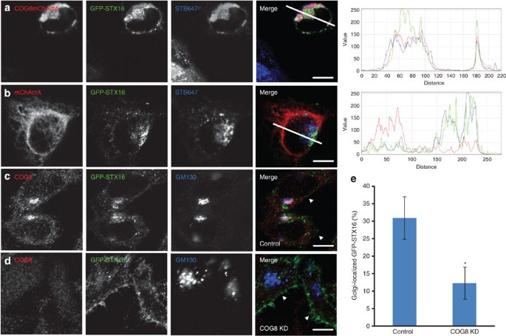Figure 7: COG8 is required for localization of STX16-containing trafficking intermediates. HeLa cells were co-transfected with plasmids encoding COG8-mChActa and GFP-STX16 (a), or mChActA and GFP-STX16 (b). Twenty-four hours after transfection, cells were pulsed with Alexa647 labelled STB (STB-647) for 20 min, then washed and additionally chased in fresh media for 2 h. Cells were fixed and analysed by confocal microscopy. HeLa cells were transfected with GFP-STX16 (c) or co-transfected with GFP-STX16 and COG8 siRNA (d) by electroporation. After 72 h, cells were fixed, stained with COG8 and GM130 antibodies and analysed using confocal microscopy. White arrows indicate change in localization of GFP-STX16 from GM130-labelled Golgi membranes to the plasma membrane. Quantitative analysis (e) performed as follows; Controln=24, COG8 KDn=31. Error bars represent s.d. STX16 fluorescence was measured using ImageJ software and measuring GFP-STX16 signal in GM130-labeled Golgi regions of interest and around the total cell. Student’st-test was used to calculateP-value. *P=4.86E-18. Scale bar, 10 μm. Figure 7: COG8 is required for localization of STX16-containing trafficking intermediates. HeLa cells were co-transfected with plasmids encoding COG8-mChActa and GFP-STX16 ( a ), or mChActA and GFP-STX16 ( b ). Twenty-four hours after transfection, cells were pulsed with Alexa647 labelled STB (STB-647) for 20 min, then washed and additionally chased in fresh media for 2 h. Cells were fixed and analysed by confocal microscopy. HeLa cells were transfected with GFP-STX16 ( c ) or co-transfected with GFP-STX16 and COG8 siRNA ( d ) by electroporation. After 72 h, cells were fixed, stained with COG8 and GM130 antibodies and analysed using confocal microscopy. White arrows indicate change in localization of GFP-STX16 from GM130-labelled Golgi membranes to the plasma membrane. Quantitative analysis ( e ) performed as follows; Control n =24, COG8 KD n =31. Error bars represent s.d. STX16 fluorescence was measured using ImageJ software and measuring GFP-STX16 signal in GM130-labeled Golgi regions of interest and around the total cell. Student’s t -test was used to calculate P -value. * P =4.86E-18. Scale bar, 10 μm. Full size image STX16 trafficking is severely affected in COG8-deficient cells STX16 is known to cycle between the TGN, endosomal membranes and the plasma membrane [24] , [25] , [26] . If COG8 has a role in localization of STX16 vesicles, we would expect that STX16 trafficking would be disrupted in COG8-deficient cells. In wild-type HeLa cells, GFP-STX16 partially colocalizes with COG8- and GM130-positive Golgi membranes, and is also present on multiple puncta that are likely to represent endosomal compartments ( Fig. 7c and Supplementary Fig. S4f ). Strikingly, in COG8-depleted cells, the majority of GFP-STX16 was found to relocalize to the plasma membrane ( Fig. 7d ), supporting the hypothesis that COG8, and possibly the whole COG Lobe B sub-complex, serves as a specific spatial landmark for STX16-carrying trafficking intermediates at the Golgi. Similarly, in COG8-deficient human fibroblasts, endogenous STX16 was mislocalized from Golgi membranes ( Supplementary Fig. S16 ) The CATCHR sub-family of multi-subunit protein complexes has long been implicated in tethering of membrane-trafficking intermediates at different steps of the secretory pathway [3] , but the exact mechanism by which these complexes orchestrate vesicular approach, recognition, tethering and fusion is still unclear. SNAREs are the major partner protein family for all CATCHR complexes [15] , [16] , [27] , [28] , [29] , and subsequently, it was proposed that one of the evolutionarily conserved functions of vesicle-tethering complexes is to assist and/or stabilize SNARE complex formation. Indeed, the steady-state levels of assembled SNARE complexes was found to be significantly lower in cells deficient of COG complex subunits [15] , [16] . In this work, we have discovered several additional SNARE partners for the Golgi-localized COG complex. In addition to the Qa SNARE STX5, previously shown to interact with COG4 and COG6 [15] , we have now discovered that the STX5 partner SNARE GS27 binds to both COG6 and COG8. These data suggest a role for the whole functional COG complex in the regulation of the cis -Golgi-localized STX5 SNARE complex. Our data also demonstrated that the TGN Qa SNARE STX16 and its partner STX6 undergo specific protein–protein interactions with COG8 and COG6, implicating Lobe B of the COG complex in regulation of the STX16-centred TGN SNARE complex. These results were not limited to the HeLa cell model, as the COG4 recruitment of STX5 vesicles and the COG8 recruitment of STX16 vesicles to mitochondria was also observed in Vero cells ( Fig. 6c–f ). In addition, Lobe B subunits can be specifically cross-linked to the endogenous STX16 ( Supplementary Fig. S17 ), further supporting the Lobe B–STX16 interaction data. Yet, another Golgi SNARE, SNAP29, was shown to interact with COG6, and to a lesser extent with COG8 and COG4 ( Fig. 1 and Supplementary Figs S1 and S2 ). SNAP29 binds to STX6 (ref. 30 ) [30] , forming a complex that is distinct from the well-studied STX16/STX6/Vti1/VAMP4 SNARE assembly, suggesting that COG may regulate an additional SNAP29/STX6-containing SNARE complex. In support of this hypothesis, it was recently found that both SNAP29 and COG physically interact with the BLOC1 complex that is responsible for specialized cargo sorting in the endosome-to-Golgi retrograde trafficking pathway [31] . The exact nature of the COG–SNARE interactions (and CATCHR–SNARE interactions in general) is still under intense investigation. These interactions likely represent a multistep regulatory cascade in which different COG subunits simultaneously, and/or sequentially, interact with individual SNARE proteins and SNARE complexes before and during SNARE complex assembly. In vitro reconstitution experiments clearly demonstrate that target-to-target (t-t) SNARE sub-complexes are formed before the fusogenic trans vesicle-to-target (v-t) SNARE complexes [32] , [33] . In this respect, the ability of different COG subunits to interact with different t-SNARE proteins may directly facilitate formation of t-t SNARE sub-complexes. For instance, simultaneous COG4-STX5 and COG6-GS27 interactions may facilitate the assembly of the STX5-GS27 intra-Golgi t-t SNARE subcomplex, whereas the concurrent COG8-STX16 and COG6-STX6 interactions would promote formation of the STX16-STX6 TGN t-t SNARE complex. In addition, the ability of different COG subunits to interact with the same SNARE protein may assist in the assembly of multiple SNARE complexes. It has been suggested that fusion of transport vesicles with target membranes is achieved by the simultaneous assembly of several SNARE complexes [34] , [35] . Therefore, the ability of several COG subunits to interact with the same Qa SNARE (for instance, COG4, COG6 and COG8 with STX5) may facilitate the synchronized formation of a fusogenic array of SNARE complexes. The most astonishing aspect of our studies is the finding that COG4 and COG8 proteins could specifically relocalize two different classes of SNARE-carrying trafficking intermediates in vivo . If transplanted to the outer mitochondria membrane, COG4 specifically attracts STX5-containing carriers, whereas COG8 prefers vesicles with STX16. To our knowledge, this is the first example of the in vivo redirection of intra-Golgi-trafficking carriers to other non-secretory cellular organelles. This unusual COG-dependent relocalization of Qa SNAREs to mitochondria could be achieved by several possible scenarios. In the first scenario (a direct protein relocalization model), the co-expressed COG and SNARE partners could form a stable pair, before membrane insertion, which would be subsequently delivered to mitochondria. Indeed, direct COG–SNARE interactions were found to be essential for the efficient co-localization of proteins. However, these protein–protein interactions were not sufficient for relocalization of STX16 vesicles to mitochondria populated with COG8 truncation mutants that were competent in STX16 binding ( Fig. 4g ). Rapid redistribution of SNARE-containing vesicles to mitochondria observed in cell fusion experiments similarly indicate that redirected vesicular trafficking is the major cause of SNARE relocalization. In the second scenario (an ER–mitochondria handshake model), newly synthesized ER SNARE proteins could be engaged in direct protein–protein interactions with the mitochondria-anchored COG subunit, bringing the ER in a very close proximity to the mitochondrial membranes. Indeed, ER–mitochondria connections are well described [36] , [37] , [38] , but we do not think that this scenario is having a leading role in the COG-induced relocalization of membranes enriched in Golgi Qa SNAREs. ER-located protein disulfide isomerase (PDI) does not generally colocalize with mitochondria-diverted GFP-STX5 or GFP-STX16 ( Supplementary Fig. S18 ). In addition, we did not detect any co-localization between CFP-STX5 and GFP-Mff, the molecule that is specifically localized in ER–mitochondria contact sites [38] ( Supplementary Fig. S18 ). Finally, in cells that overexpress CFP-GalT, only the Golgi pool of CFP-GalT was found in a vicinity of COG4-bearing mitochondrial aggregates ( Supplementary Fig. S19 ), whereas the ER-localized pool of GalT-CFP [39] was not disturbed. Most importantly though, the relocalization of SNARE-containing vesicles to mitochondria was regulated by the same components that were previously implicated in ‘normal’ intra-Golgi trafficking. STX16 redirection to COG8-mitochondria was inhibited by overexpression of Vps45 ( Fig. 4g ), whereas recruitment of STX5 vesicles to COG4-mitochondria required the presence of other COG subunits and participation of Sly1p ( Supplementary Fig. S9 ). In addition, STX5 recruitment to COG4-mitochondria was partially inhibited by Brefeldin A treatment ( Supplementary Fig. S20 ). All these factors indicate the active involvement of coat protein complex I (COPI)-mediated vesicular trafficking in the relocalization process. Strikingly, in cells that express a modest level of COG4-mChActA, GFP-STX5 was mostly localized in vesicle-like punctate structures along the mitochondrial membranes (data not shown). Similar vesicular profiles were found in close proximity to mitochondrial membranes in TEM and Immuno-EM images ( Fig. 6 ), suggesting a third relocalization scenario (a vesicle re-routing model), in which mitochondria-localized COG subunits serve as vesicle-tethering platforms that are sufficient for capturing specialized classes of membrane-trafficking intermediates. The COG4 platform includes other protein subunits from both Lobe A and Lobe B sub-complexes, whereas the COG8 platform is mostly enriched in Lobe B subunits. The two different COG platforms showed striking specificity for capturing either STX5 (COG4 platform) or STX16 (COG8 platform) containing vesicular carriers. STX5 vesicles were enriched in the ER–Golgi recycling marker ERGIC53 ( Supplementary Fig. S21 ), and are likely to represent cis /medial Golgi recycling carriers. On the other hand, STX16 vesicles partially co-localized with endocytosed Shiga toxin, and most likely represent endosome-to-Golgi recycling carriers ( Fig. 7a ). We favour this latter vesicle relocalization scenario; however, the exact mechanism by which Qa SNARE-carrying transport intermediates are diverted to mitochondria will require additional investigation. How can the data from the mitochondria relocalization assay be interpreted with regard to COG complex function in Golgi trafficking? We propose that, in addition to the direct facilitation of SNARE complex assembly, the essential function of the COG complex is to serve as a spatial landmark for the localization of Qa SNAREs within Golgi subdomains. In this model, the complete COG complex determines the location of the cis /medial Qa SNARE STX5, whereas the Lobe B COG subcomplex, which exists as a separate entity in both soluble and membrane-bound forms, determines the position of the trans Qa SNARE STX16 ( Fig. 8 ). In support of this hypothesis, we found that STX16 is severely mislocalized in cells deficient for COG8 ( Fig. 7e ). This SNARE-positioning function is likely to be conserved for all multi-subunit tethering complexes. 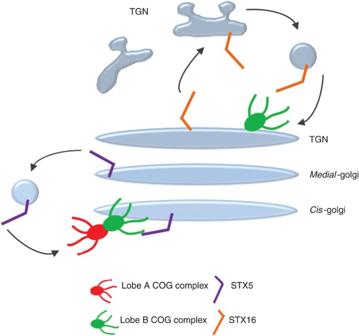Figure 8: COG complex serves as a spatial landmark for precise localization of Qa SNAREs in Golgi subdomains. Hypothetical model of how the COG complex functions in organizing different SNARE complexes on Golgi membranes. The recycling STX5-containing SNARE complex (purple rod) is targeted by both lobe A and lobe B of the COG complex to direct it tocis-Golgi membranes. The TGN-localized STX16-containing SNARE complex (orange rod) is targeted by lobe B of the COG complex to direct it to TGN membranes. Figure 8: COG complex serves as a spatial landmark for precise localization of Qa SNAREs in Golgi subdomains. Hypothetical model of how the COG complex functions in organizing different SNARE complexes on Golgi membranes. The recycling STX5-containing SNARE complex (purple rod) is targeted by both lobe A and lobe B of the COG complex to direct it to cis -Golgi membranes. The TGN-localized STX16-containing SNARE complex (orange rod) is targeted by lobe B of the COG complex to direct it to TGN membranes. Full size image In light of this model, there are numerous questions to be resolved, such as how the COG complex localizes itself onto Golgi subdomains, and are there major receptors for COG sub-complexes on the Golgi? These are crucial questions for future investigations. The development of the mitochondrial relocalization assay provides an excellent tool to address the biochemical requirements of the COG-mediated vesicle-tethering process in vivo . Reagents and antibodies Protein G agarose were from Roche. Antibodies used for IF microscopy or western blotting (WB) were purchased through commercial sources, gifts from generous individual investigators or generated by us via affinity purification. Antibodies were as follows: Rabbit polyclonal: Myc (Bethyl Laboratories); COG3, COG4, COG6, COG8 (this lab); GS27 (Synaptic Systems); Giantin (Covance); TGN46 (AbD Serotech). Mouse monoclonal: GFP (Molecular Probes); GFP (Covance); GM130 (BD Biosciences); p115; GPP130 (Alexis); PDI (Affinity BioReagents); ERGIC53 (Enzo Life Sciences); Ox Phos ComplexV (Invitrogen); and Myc (Cell Signaling). Secondary IRDye 680 goat anti-rabbit, IRDye 700 goat anti-mouse and IRDye 800 donkey anti-goat for WB were from LI-COR Biosciences. Anti-rabbit HiLyte 488, HiLyte 555 and DyLight647 for IF were obtained from AnaSpec and Jackson ImmunoResearch, Inc. Cell culture HeLa cells were cultured in DMEM/F-12 medium (Thermo Scientific) supplemented with 15 mM HEPES, 2.5 mM L -glutamine and 10% FBS (Atlas Biologicals) at 37 °C and 5% CO 2 in a 90% humidified incubator. GFP-COG6 stable cell lines were generated by transfecting cells with pEGFP-C1-COG6 followed by selection for G418 resistance in complete medium supplemented with 0.4 mg ml −1 G418 sulphate. YFP-COG3 stable cell lines were generated as described [15] . siRNA-induced knockdowns siRNA duplexes for COG1 (D-013309-01 (5′-UAGAUGACCUCCUGGCUUA-3′) and D-013309-04 (5′-GUAGCGGCCUCUCCAUGAA-3′)), COG2, COG3, COG4 and COG8 [12] , [21] , [23] were obtained from Dharmacon (Chicago, IL). Transfection was performed using lipofectamine RNAiMAX siRNA Transfection Reagent (Invitrogen) and cells were analysed 72 h after transfection. Plasmid preparation and transfection Yeast and mammalian-expression constructs were generated using standard molecular biology techniques or obtained as generous gifts ( Supplementary Table 1 ). cDNA constructs expressing SNAREs were from Open Biosystems. DNA fragments encoding cytoplasmic domains of SNAREs were subcloned into pGBDU vector as Eco R1/ Sal 1 or Bgl II/ Xho 1 inserts and verified by sequencing. Human COG8 with deletions of aa 8–148 and 8–436 were generated by PCR using hCOG8-pEGFP as a template. hCOG1 (898–980) was generated by PCR and subcloned into pCDNA3.1 ( Bam HI/ Xho 1). To generate fluorescently tagged chimeras full-length, proteins were inserted into pECFP-C1, pEGFP-C1 ( Bsp E1/ Bam HI) or pmCherry-C1-ActA ( Bsp E1/ Nde I) vectors. pEGFP-C1-STX16 deletions aa 2–73 or 2–169 were generated by PCR using pEGFP-C1-STX16 as a template. To generate STX5-mChActA and STX16-mChActA, cytoplasmic domains of rSTX5a and hSTX16 were amplified by PCR and subcloned into pmCherry-C1-ActA vector. Plasmids were isolated from bacterial cells using the QIAprep Spin Miniprep Kit (Qiagen). Plasmid transfections into tissue culture cells were performed with Lipofectamine 2000 (Invitrogen). IF microscopy Cells were grown on glass coverslips 1 day before transfection. After transfection, cells were fixed and stained as described previously [12] . Cells were imaged with the X63 oil 1.4 numerical aperture (NA) objective of a LSM510 Zeiss Laser inverted microscope outfitted with confocal optics. Image acquisition was controlled with LSM510 software (Release Version 4.0 SP1). The ‘RGB profiler’ plug-in of Image J ( http://rsbweb.nih.gov/ij ) was used to generate line plots for individual channels. The ‘Coloc_2′ plug-in was utilized to calculate Pearson’s coefficient for co-localization. At least three independent experiments were performed to calculate both mean and s.d. values. SDS–PAGE and WB SDS–PAGE and WB were performed as previously described [14] . Blots were incubated with primary antibodies, and then with a secondary antibody conjugated with IRDye 680 or IRDye 800 dyes. Blots were scanned and analysed with an Odyssey Infrared Imaging System (LI-COR Biosciences). At least three independent experiments were performed to calculate both mean and s.d. values. Yeast two-hybrid assay The following constructs were used in yeast two-hybrid assay: COG subunits (1–8) of mammalian COG complex were cloned as C-terminal fusion constructs with Gal4 AD, and SNARE constructs lacking transmembrane domain were cloned as C-terminal fusion constructs with Gal4 BD by recombination cloning in yeast. The Gal4 two-hybrid system was used as described [18] , [40] . Reporter strains of opposite mating types were transformed with bait and prey fusion constructs. Growth of independent transformants was assessed on media lacking leucine (prey fusions) and uracil (bait fusions). Diploid yeasts containing combinations of the human COG subunits 1–8 and SNAREs, as well as empty vectors and pair-wise combinations of human COG2/4 (ref. 11 )), were created by mass mating. Yeast diploids were selected on −LEU/−URA plates. Diploids were grown in liquid −LEU/−URA medium to the same optical density (D600=0.8) and titrated 1:10, 1:100, 1:1,000 and 1:10,000 in ddH 2 O. A volume of 5 μl of each dilution was applied on a selective medium lacking adenine, histidine and leucine/uracil, incubated at 30 °C for 72 h and scored for growth. Expression of all hybrid molecules was verified by WB. The relative stringency of direct protein–protein interaction was estimated by growth assay on agar plates lacking either histidine (−HIS; leaky regulation) or adenine (−ADE; high stringency regulation). Immunoprecipitations Cells were collected and lysed in a 1% Triton X-100 PBS buffer with 10 μl ml −1 of 100 × Halt protease inhibitor cocktail for 1 h on ice. Post-nuclear supernatant was cleared and 90% was added to GFP antibodies and incubated on ice overnight. Next day, protein G agarose beads (Roche) was added to each reaction, and samples were incubated at 4 °C on a rotator for 2 h. Unbound material was removed, beads were washed 4 × in 0.05% Triton X-100 in PBS and eluted in 2 × sample buffer. Fluorescence recovery after photobleaching HeLa cells grown on glass-bottom culture plates were transiently transfected with COG8-mChActA and GFP-STX16 plasmids. Fluorescence recovery after photobleaching was performed using a laser-scanning confocal microscope (LSM 710 Zeiss Laser inverted microscope outfitted with confocal optics) equipped with an environmental control system (Live cell system; Biovision Technologies) set to 37 °C and 5% CO 2 . Cells were cultured in phenol red-free DMEM/F-12 (Sigma-Aldrich) with 1% FBS. Pre-bleached images were taken for 12 s (7 s per frame), and the selected mitochondria area was bleached for 5 s using a pulse of the 488- and 561-nm laser lines at maximal intensity and 15 iterations/regions of interest. After bleaching, fluorescence images were then recorded every 7 s for 6 min 45 s. Transmission Electron Microscopy Samples were treated according to Valdivia’s lab protocol [41] with modifications. In short, cells were fixed for 20 min on ice with 2.5% glutaraldehyde and 0.05% malachite green (EMS) in 0.1 M sodium cacodylate buffer, pH 6.8. Samples were post-fixed for 30 min at room temperature (RT) with 0.5% osmium tetroxide and 0.8% potassium ferricyanide in 0.1 M sodium cacodylate, for 20 min on ice in 1% tannic acid, and for 1 h in 1% uranyl acetate at RT. Specimens were dehydrated with a graded ethanol series and embedded in Araldite 502/Embed 812 resin (EMS). Ultrathin sections were imaged at 80 kV on a FEI Technai G2 TF20 TEM and images were acquired with a FEI Eagle 4kX USB Digital Camera. Immuno-electron microscopy Vero cells were co-transfected with COG4-mChActA and GFP-STX5. 20 h after transfection cells were washed in PBS and fixed in 4% paraformaldehyde for 30 min. After washing in 50 mM NH 4 Cl in PBS for 5 min, cells were blocked in 1% BSA, 0.1% saponin in PBS solution twice for 10 min at RT. Cells were exposed to rabbit anti-GFP antibodies (1:500) in 1% fish gelatin, 0.1% saponin in PBS for 2 h at RT, washed in 0.005% saponin in PBS and then incubated with the Fab’ fragment of a goat anti-rabbit IgG conjugated to colloidal gold (1.4 nm in diameter; Nanoprobes) in 0.005% saponin in PBS for 2 h. The cells were fixed in 1% glutaraldehyde in PBS for 10 min and washed in 50 mM glycine in PBS, 1% BSA in PBS and H 2 O. The gold labelling was intensified with a gold enhancement kit GoldEnhance-EM (Nanoprobes) for 2 min following the manufacturer’s protocol. After rinsing cells in 1% aqueous sodium thiosulfate and H 2 O, the cells were post-fixed in PBS containing 1% OsO 4 and 1.5% potassium ferrocyanide for 60 min, washed in H 2 O, dehydrated in a series of graded ethanol solutions and embedded in Araldite 502/Embed 812 resin (EMS). Toxin trafficking assay Cells were grown on glass coverslips 1 day before transfection. After transfection, cells were washed with cold PBS and incubated on ice with Alexa Fluor 647 labelled Shiga toxin B subunit (STB-647) or Subtilase cytotoxin (SubAB647) for 20 min. Cells were washed to remove unbound toxin and incubated with fresh media at 37 °C for 1 h. Cells were then fixed and prepared for IF staining as indicated above. Toxins were labelled according to the manufacturer’s protocol (Invitrogen). Cell fusion assay Transiently transfected Vero cells were grown on coverslips and imaged using a laser confocal spinning disk microscope system based on a Nikon TiE microscope, equipped with a Yokogawa CSU-X1 and an Andor iXon+ EMCCD camera and fitted with 40 × , 1.30 NA and 100 × , 1.49 NA objectives. Image acquisition was controlled with Andor Bioimaging software (Andor IQ2.1). After start of time-lapse image acquisition, cell–cell fusion was mediated by a HVJ envelope cell fusion kit (GenomeONE-CF EX; Cosmo Bio Co.). For cell fusion to occur, cells were washed once with 'cell fusion buffer' following the manufacturer’s protocol and incubated for 10 min with a 1:40 dilution of the HVJ envelope solution, leading to efficient fusion of cells contacting each other. How to cite this article: Willett, R. et al . COG complexes form spatial landmarks for distinct SNARE complexes. Nat. Commun. 4:1553 doi: 10.1038/ncomms2535 (2013).